Morphology and mixing state of individual freshly emitted wildfire carbonaceous particles Biomass burning is one of the largest sources of carbonaceous aerosols in the atmosphere, significantly affecting earth’s radiation budget and climate. Tar balls, abundant in biomass burning smoke, absorb sunlight and have highly variable optical properties, typically not accounted for in climate models. Here we analyse single biomass burning particles from the Las Conchas fire (New Mexico, 2011) using electron microscopy. We show that the relative abundance of tar balls (80%) is 10 times greater than soot particles (8%). We also report two distinct types of tar balls; one less oxidized than the other. Furthermore, the mixing of soot particles with other material affects their optical, chemical and physical properties. We quantify the morphology of soot particles and classify them into four categories: ~50% are embedded (heavily coated), ~34% are partly coated, ~12% have inclusions and~4% are bare. Inclusion of these observations should improve climate model performances. Biomass burning (BB) emissions significantly impact radiative forcing of climate at regional and global scales [1] . Global annual emissions of black carbon (BC) and organic carbon (OC) aerosols are estimated as ~8 and 33.9 Tg yr –1 , respectively, and the contributions from open burning are estimated as 42% for BC and 74% for OC [2] . However, current estimates of BB emissions are highly uncertain (a factor of 3–5 for individual aerosol and gaseous species) [3] . In addition, the emission of BB carbonaceous aerosols could increase, as future global and regional warming accentuate favourable conditions for wildfire activities [4] . A recent study shows that the radiative forcing from BB can vary non-linearly with the concentration of co-emitted trace gases and aerosols [5] . BB aerosol is estimated to have a highly uncertain net positive direct radiative forcing (for example, 0.03±0.12 W m −2 in IPCC [6] and Myhre et al. [7] ). Recently, Bond et al. [3] estimated the direct radiative forcing from the total BC burden as +0.71 W m −2 (with 90% uncertainty bounds from +0.08 to 1.27 W m −2 ). They also estimated the contributions from open burning as +0.20 W m −2 (with 90% uncertainty bounds from −0.50 to +1.08 W m −2 ). The uncertainty is due to many factors including the balance between a large positive forcing by BC and a large negative forcing by OC. Mixing state and composition of the aerosols can strongly influence the balance of radiative forcing by BC and OC. Models estimate an enhancement of BC forcing up to a factor of 2.9 when BC is internally mixed with other aerosols, compared with externally mixed scenarios [8] . Internal mixing of BC emitted from BB might enhance absorption by 70%, with OC coatings having a key role [9] . In contrast, a recent study on urban plumes suggests that the aerosol absorption enhancement for mixed BC might have been overestimated in models [10] . It is unclear how these findings might apply to other BC sources including BB. Following the contrasting results of these and similar studies, there is an intense debate about the issue of absorption enhancement, the appropriateness of scaling point measurements up to scales relevant to global climate models, and conversely, the ability of models to correctly capture the enhancement in different environments [10] , [11] , [12] . To add to the debate, recently, there has been a renewed discussion about what the term ‘BC’ really means [13] , [14] . In addition to the BC mixing state issue, the optical and physical properties of tar balls (TBs) that constitute a large fraction of the total BB aerosols are highly uncertain [15] , [16] , [17] . Electron microscopy has been used widely to investigate BB particles size, morphology, chemical composition and mixing state. These parameters can vary largely depending on aerosol sources, formation temperature, transport, condensation and evaporation of primary and secondary gases [18] , [19] , [20] , [21] . In this study, we report a detailed analysis of a large number of single BB particles from the Las Conchas fire. We discuss coating and oxidation of TBs and morphological properties of aggregates of carbonaceous nanospheres and their mixing with other materials. We refer to aggregates of carbonaceous nanosphere particles as soot. As we analyse particles only from BB combustion, we consider soot to well represent BC in BB smoke. As described in the Methods section, we used a thermodenuder to remove most of the volatile compounds from the BB aerosols, and in the following sections we describe the differences in the properties of ambient versus thermodenuded particles to understand coating effects. We report the existence of two distinct types of TBs, which differ in their degree of oxidation and coating. We also classify soot particles based on their coating and morphology and discuss their properties. Aerosol from BB is still poorly characterized and these findings should improve our understanding of atmospheric processing of BB aerosols and their effects on climate. Particle classification Based on morphology and elemental composition, we classified over 4,200 particles into three categories: TBs, soot and others particles. The classification is similar to that adopted by Adachi and Buseck [22] except that we combined organic matter and irregularly shaped particles as dust and salt, in the ‘other’ category. We also want to underline that the category ‘soot’ includes soot particles that are coated by other material, as further discussed later. TBs are amorphous, spherical carbonaceous particles that show no crystallographic structure and normally are most abundant in slightly aged (minutes to hours) BB smoke [20] . TBs are easily identified because of their spherical shape and resistance to electron beam damage [19] . Energy-dispersive X-ray spectroscopy (EDS) of our samples shows that TBs are mainly composed of C and O, and sometimes contain traces of K and S. It is believed that TBs are similar to high-molecular weight humic-like substances formed during gas to particle phase transitions, involving rapid polymerization of lignin products induced by OH radicals [18] , [20] , [23] . In contrast, fresh soot exhibits a characteristic chain-like morphology as agglomerates of small spherical monomers [13] . The soot particles investigated here are often mixed with other organic and inorganic material also emitted by fire [24] . Ambient samples (denoted in this paper as A-1 and A-2) had an average of 80% TBs by number with an average of 8% soot and 12% of other particles. The fraction of TBs is similar to other studies [18] , [20] , [21] where fractions up to 90% have been reported, although a lower fraction of TBs (~15%) have been found for relatively fresh samples (within a few minutes of aging) [22] . Identification of two kinds of TBs Using secondary electron (SE) imaging of individual particles at low accelarating voltage (1 kV) [25] , we identified two distinct kinds of TBs, ‘electronically’ dark and bright ( Fig. 1a ), whereas TBs appear indistinguishable at high accelerating voltage (10 kV) ( Fig. 1b ). We conjecture that the enhanced contrast at low accelerating voltages is due to different SE yields owing to various degree of oxidation at the particle’s surface. A similar SE contrast effect has been observed on zinc versus zinc oxide samples [25] . However, estimation of SE yields for individual TBs is complicated because of their complex and uncertain composition and mixing. In addition to SE imaging, we imaged the TBs in our samples using backscattered electrons (BSEs) and found no prominent contrast difference between the two types of TBs. Typically, detected SEs originate from very small escape depths (a few nanometres deep within the sample), much smaller than the dimensions of the particles, whereas BSEs are detected even when generated from relatively large depths (10–100 s of nm), which are comparable to the particle size [26] . In other words, SEs are sensitive to the surface, whereas BSEs are sensitive to the bulk of the particle. Tivanski et al. [23] found a 40-nm thick oxygenated interface layer around the TBs after atmospheric processing. The fact that we found different contrasts in the SE images, but not in the BSE images, is consistent with the existence of a layer of different composition at the surface of the TBs. 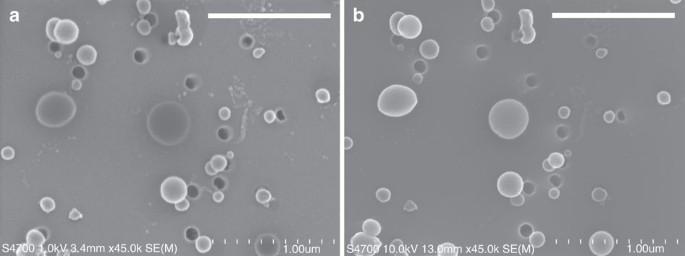Figure 1: Identification of electronically dark and bright spherical TB particles. Field-emission scanning electron microscopy micrographs of ambient particles collected from the Las Conchas fire. (a) Image at low working distance (3.4 mm) and low accelerating voltage (1 kV). (b) Image of the same particles, but at higher working distance (13 mm) and higher accelerating voltage (10 kV). Electronically bright and dark TBs are evident at the low accelerating voltage, but not at the high accelerating voltage. Scale bars, 1 μm. Black circles are pores in the nucleopore filter. Figure 1: Identification of electronically dark and bright spherical TB particles. Field-emission scanning electron microscopy micrographs of ambient particles collected from the Las Conchas fire. ( a ) Image at low working distance (3.4 mm) and low accelerating voltage (1 kV). ( b ) Image of the same particles, but at higher working distance (13 mm) and higher accelerating voltage (10 kV). Electronically bright and dark TBs are evident at the low accelerating voltage, but not at the high accelerating voltage. Scale bars, 1 μm. Black circles are pores in the nucleopore filter. Full size image We classified ‘electronically’ dark and bright TBs based on their grayscale intensity on the SE low-accelerating voltage SEM images ( Supplementary Fig. S1 ). We found that approximately 32% of the TBs are dark in ambient samples. 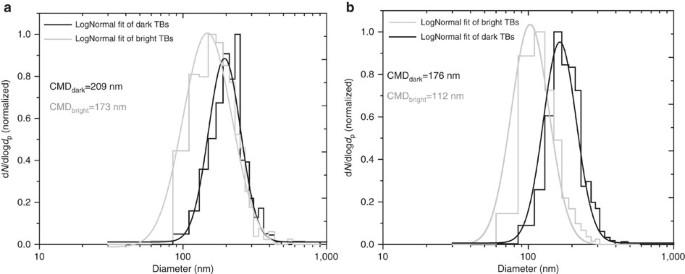Figure 2: Size distribution of ambient- and denuded-bright and -dark TBs. Size distribution and lognormal fits of: (a) ambient particles (435 dark and 930 bright particles); (b) denuded particles (415 dark and 1,086 bright particles). The number of particles in each size bin is normalized by the bin width in logarithmic space, and the mode of the distribution is normalized to 1. The light grey lines represent bright TBs and the dark lines represent dark TBs. The difference between the count median diameter for ambient-dark and denuded dark TBs is 33 nm (209−176 nm), whereas the difference between ambient-bright and denuded-bright TBs is 61 nm (173−112 nm). Dark TBs display smaller reduction in size on denuding, consistent with being more refractory. Figure 2a shows the size distributions of ambient TBs and denuded TBs, respectively. Dark and light grey lines represent the lognormal fit of dark and bright TBs, respectively. Dark TBs are larger in both ambient and denuded samples. The difference between the size of ambient-bright and denuded-bright TBs (61 nm) is larger than the difference between the size of ambient-dark and denuded-dark TBs (33 nm), implying that on average more material was removed by the denuder for bright TBs. This could indicate thicker coating and/or coating material having different volatility. Figure 2: Size distribution of ambient- and denuded-bright and -dark TBs. Size distribution and lognormal fits of: ( a ) ambient particles (435 dark and 930 bright particles); ( b ) denuded particles (415 dark and 1,086 bright particles). The number of particles in each size bin is normalized by the bin width in logarithmic space, and the mode of the distribution is normalized to 1. The light grey lines represent bright TBs and the dark lines represent dark TBs. The difference between the count median diameter for ambient-dark and denuded dark TBs is 33 nm (209−176 nm), whereas the difference between ambient-bright and denuded-bright TBs is 61 nm (173−112 nm). Dark TBs display smaller reduction in size on denuding, consistent with being more refractory. Full size image Semi-quantitative EDS was conducted on 25 dark and 25 bright TBs of comparable size. Out of the 25 dark TBs, 18 showed higher average oxygen content (50 atomic %) than in bright TBs (35 atomic %) ( Supplementary Fig. S2 ). The remaining seven dark TBs showed similar oxygen content to the bright TBs possibly due to the presence of an insulating layer or due to the somewhat subjective segregation of each TB group. Similarly, Tivanski et al. [23] found that TBs consist of 55% atomic carbon and 45% atomic oxygen and, as mentioned earlier, suggested the existence of an oxygenated layer on TBs. This analysis, together with the comparison of the size distribution of denuded versus ambient TBs (dark TBs display smaller reduction in size upon denuding than bright TBs do), suggests that the dark TBs are more oxidized and possibly have a less volatile coating. 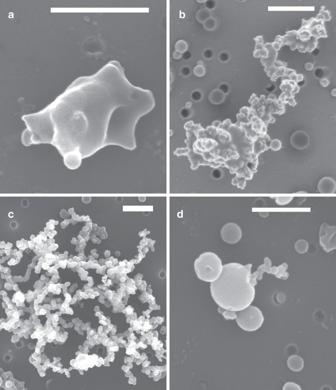Figure 3: Mixing and classification of soot particles. Field-emission scanning electron microscope images of four different categories of soot particles: (a) embedded, (b) partly coated, (c) bare and (d) with inclusions. Approximately 50% of the ambient soot particles are embedded, 34% are partly coated and 12% have inclusions. Only 4% of the particles are bare soot (not coated or very thinly coated). Scale bars, 500 nm. Mixing of soot particles Figure 3 shows an example of soot particles from the Las Conchas fire classified into four categories based on morphology and visual estimation of coating: (a) embedded soot, where the particle is heavily coated [27] (potentially corresponding to a large optical absorption enhancement), but where some monomers are still evidently visible; (b) partly coated, where soot voids are filled by coating material, but the soot is not completely engulfed; (c) bare soot, where monomers are easily distinguished and no considerable coating is evident from the SEM image, although very thin coating might be present on the monomers (corresponding to no or little optical absorption enhancement); (d) soot with inclusions, where soot is mixed with, but not uniformly coated by, other material or particles. Of the 1,026 soot particles analysed, 50% were heavily coated, 34% partly coated, 4% bare and 12% with inclusions. We should caution that the count of embedded soot particles might be biased low because when the coating is very thick, the monomers of the soot particle might not be distinguishable, and then the particle would not be classified as soot. Figure 3: Mixing and classification of soot particles. Field-emission scanning electron microscope images of four different categories of soot particles: ( a ) embedded, ( b ) partly coated, ( c ) bare and ( d ) with inclusions. Approximately 50% of the ambient soot particles are embedded, 34% are partly coated and 12% have inclusions. Only 4% of the particles are bare soot (not coated or very thinly coated). Scale bars, 500 nm. Full size image Morphology of ambient and denuded soot particles Soot particles are ‘fractal-like aggregates’ and their ensemble morphology can be characterized by analysing many individual aggregates using the following statistical scaling law [28] : where N is the number of monomers per aggregate, R g is the radius of gyration of the aggregate, d p is the monomer diameter, k g is called fractal prefactor and D f is the mass fractal dimension. For a given D f , k g represents the level of compactness, with a smaller prefactor indicating lower packing [29] . 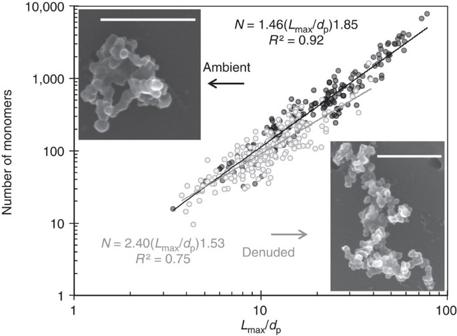Figure 4: Fractal dimension of soot particles. Fractal dimension of ambient-1 (in black) and denuded-1 (in grey) soot particles. The fractal dimension of ambient and denuded soot is 1.85±0.05 (n=176) and 1.53±0.07 (n=209), respectively. s.e. was calculated from the uncertainty in the mean‐square fit considering the uncertainty inNanddp. The insets provide examples of ambient-1 and denuded-1 soot particles. Scale bars, 500 nm. Figure 4 shows an example of the estimation of the fractal dimension of soot particles for ambient-1 and denuded-1 samples. The details of the calculation are provided in the Methods section ( Supplementary Table S1 ). Figure 4: Fractal dimension of soot particles. Fractal dimension of ambient-1 (in black) and denuded-1 (in grey) soot particles. The fractal dimension of ambient and denuded soot is 1.85±0.05 ( n =176) and 1.53±0.07 ( n =209), respectively. s.e. was calculated from the uncertainty in the mean‐square fit considering the uncertainty in N and d p . The insets provide examples of ambient-1 and denuded-1 soot particles. Scale bars, 500 nm. Full size image For completeness, we estimated three other morphological descriptors: aspect ratio, roundness and area equivalent diameter ( D Aeq ) [30] . In Table 1 , we summarize all the morphological descriptors for ambient (A-1 and A-2) and corresponding denuded (D-1 and D-2) particles collected during two different time periods. Table 1 Morphological descriptors of soot particles. Full size table As expected, for both samples, D f is larger for ambient than denuded particles. Different organic and inorganic substances can condense on soot particles [21] ; this coating is partially removed during the denuding process, resulting in smaller particles with less-filled voids and therefore lower D f . The conceptual model is that the D f of denuded soot particles represents the morphology of the soot particles as they are stripped of most of the volatile coating. What is left after denuding might or might not represent the nascent soot immediately after formation depending on the atmospheric processing. In fact, the coating material might actually modify the morphology of the soot core by rearranging the monomers position before the aerosol reaches the sampling location. The reduction in particle size after denuding is evident by noting that D Aeq decreased by 46% and 40% for sample-1 and sample-2, respectively. The values of d p (42–56 nm) are within the range (20–60 nm) of previous studies [19] and decreased by up to 20% after denuding. The higher maximum length, L max , and the higher d p in the ambient samples result in higher estimates of N and D f . Filling of the voids by condensed material on ambient particles results in more compact (higher roundness) particles ( Table 1 ). D f reflects the history of a fractal-like particle and is controlled by source, combustion conditions and aging processes [28] . Densely packed or compacted soot particles have higher D f than chain-like branched clusters or open structures [31] . Compaction of aggregates due to coating contributes to changes in particle size and D f . In a previous laboratory study, the mass-mobility exponent, which is equivalent to D f , of coated soot was found to be higher than for denuded and nascent soot [32] . The level of compaction depends on the coating material due to surface tension forces, discharge of electrostatic forces [32] and/or capillary forces acting on aggregate chains during the condensation–evaporation cycle [29] . In our study, the D f of three soot types was investigated separately: highest D f was found for embedded soot followed by partly coated and bare soot; although denuded soot did not show a similar pattern ( Supplementary Figs S3 and S4 ), possibly due to restructuring of the soot particles by the denuding process. The changes in D f for embedded particles (Δ D f(embedded) =D f(ambient) − D f(denuded) ) are statistically significant for both samples, Δ D f(embedded) =0.42±0.17 ( P =0.01, paired Student’s t -test) and Δ D f(embedded) =0.34±0.16 ( P =0.03, paired Student’s t -test) for sample-1 and sample-2, respectively. It is interesting to note that the difference between D f for all ambient and denuded soot (excluding soot with inclusions) is 0.32±0.09 and 0.18±0.08 for sample-1 and sample-2, respectively. This suggests that in general particles were more coated in sample-1 than in sample-2. The changes in morphology of the mixed particle upon denuding are also confirmed by the differences in D Aeq and L max in ambient and denuded samples. Finally, we note that for denuded-1 soot, D f (1.53) is quite smaller than for denuded-2 particles (1.74), even though the average denuder temperature was higher in the denuded-2 sample. This suggests that the structure of the denuded soot in sample-2 was more compact than in sample-1. Our analysis of the Las Conchas fire shows that approximately 32% of the TBs were highly oxidized and 50% of the soot particles were heavily coated. Increased oxidation of organic aerosol has been found to correlate with enhanced ice nucleation efficiency [33] . Similarly, the existence of different oxidation states in TBs could influence cloud condensation nuclei activity, ice nucleation and TB scavenging; this should be the subject of further study to assess the indirect effects of TBs on climate. Furthermore, the oxidation state of atmospheric particles affects their optical properties [34] , [35] in terms of their effective index of refraction and size, therefore impacting their direct effect on climate. Typically, TBs and the variability in their optical properties are not accounted for in climate models. However, recently, general circulation climate models have started including simplified schemes to account for soot mixing [8] , [36] , [37] , [38] and TBs [39] , as well on regional scales [40] . The refractive index values of TBs vary greatly in the literature and probably differ substantially for various conditions (for example, environmental conditions, location, aging and BB fuel type) [15] , [16] . Our analysis shows that the properties of TBs might be highly variable even within the same fire event. Furthermore, aerosol radiative forcing strongly depends on the description of coating and mixing state of BB particles within the models [8] , [41] . Our measurements of soot mixing state provide quantitative observational guidance on the applicability and validity of particle-resolved mixing state models [42] . These details are crucial to assess the accuracy of climate models in describing the contribution of BB aerosol radiative forcing [43] and their direct and indirect climate effects. Finally, the abundance of embedded soot particles can be used to understand the enhancement potential of (or lack thereof) absorption and scattering of internally mixed soot particles [10] , [44] . Aerosol sampling The Las Conchas wildfire started on 26 June 2011 in northern New Mexico, USA, and burned an area of 245 square miles. This was the second largest wildfire in New Mexico state history and the largest at the time. The particles were collected during the smouldering phase at a mean distance of ~25 km from the emission location (~1–2 h aged). Aerosol samples were collected on nucleopore filters (100 nm pores) at the Physics Building in Los Alamos National Laboratory during the third week of the wildfire. A thermodenuder (University of Northwest, Switzerland) was used to remove volatile compounds at temperatures up to 200 °C, leaving behind refractory soot and low-volatility compounds. We note that even at 200°C many non-refractory organic material and other inorganic coatings may still remain [11] . Two sample lines were used for collecting ambient and denuded particles with automated switching occurring at 5 min intervals. Two sets of ambient and denuded samples were collected on 12 July; the first set (ambient-1 and denuded-1) was collected from 1300 to 1720 hours, and the second set (ambient-2 and denuded-2) was collected from 1730 to 1800 hours. The denuding system was originally set up also to study the optical properties of the aerosol. To study the changes in optical properties versus the denuding temperature, the temperature during the sample-1 period was ramping from 100 to 200 °C with a mean time-weighted temperature of 152 °C. The analysis and discussion of the optical properties of the aerosols are beyond the scope of this paper, as we intentionally focus on the morphological properties. However, to accumulate enough samples for electron microscopy, aerosol was collected during the entire period and we cannot separate particles that underwent different denuding temperatures, although we can still obtain useful information on a statistical basis. On the contrary, for the denuded-2 (D-2) sample, the denuder temperature was kept constant at 200 °C. Microscopy analysis The individual aerosol particles were investigated using a field-emission scanning electron microscope (Hitachi S-4700) and EDS to distinguish different carbonaceous particles and their shape, size, elemental composition and mixing state. We used grayscale intensity to classify ‘electronically’ dark and bright TBs. Supplementary Fig. S1 shows the histogram of the grayscale intensity. The distribution of grayscale intensities ranged from 0 to 256; a threshold of 120 was selected after analysing the distribution. TBs with grayscale intensity <120 were categorized as dark and >120 were categorized as bright. Grayscale intensity for dark particles peaks between 60 and 70, whereas for bright particles peaks between 250 and 256. Supplementary Fig. S2 shows the distribution of atomic oxygen content obtained from semi-quantitative EDS analysis. EDS was conducted on 25 dark TBs and 25 bright TBs of comparable size. First, the dark and bright TBs were selected using a 1-kV accelerating voltage at 2–3 mm working distances; then the settings of the microscope were changed to 10 kV and 12 mm working distance to enable the EDS analysis. Fractal dimension analysis of soot particles The total number of monomers ( N ) in a fractal aggregate is estimated from the projected area of the aggregate ( A a ) and the mean projected area of the monomers ( A p ) in the aggregate, as follows [45] , [46] , [47] : where α is an empirical projected area exponent and k a is a constant, typically approximated with a value close to 1. To calculate N , we first estimate the overlap parameter, δ from the two-dimensional images; δ is defined as the ratio of the monomer diameter to the distance between the centres of two touching monomers [46] . We then select α and k a based on a relationship developed by Oh and Sorensen [46] , as discussed later. A caveat of this approach is that an accurate estimation of δ from two-dimensional projected images is difficult [46] . The estimated values of δ in our samples ranged from 1 (point contact) to 1.7 with median and mode of 1.5. We used α =1.13 and k a =1.50. In Oh and Sorensen [46] , the values of α and k a for a given δ are based on the assumption that the soot particles are formed via diffusion-limited cluster aggregation. However, most of the soot particles analysed in our samples are coated by organic or inorganic material, and the effect of coating might limit the validity of this approach. We therefore performed a sensitivity analysis to investigate the effects that different overlap parameters might have on the calculation of N , the fractal dimension D f and the prefactor k g . Supplementary Table S1 reports the results of this analysis for different overlap parameters ( δ =1–1.5) and for α and k a values most commonly used in literature of 1.09 and 1.15 (or 1), respectively. Images of individual soot particles were used for the calculation of the fractal dimension using equation (3): where we used the maximum length of the aggregate as an approximation for 2 R g into equation 1 as follows: L max /2 R g =1.50±0.05 (ref. 48 ). Particles categorized as ‘soot with inclusions’ were not used for the calculation of D f , as the projected area of the whole particle (including the inclusion) would bias the calculation of N and therefore D f . For the other three types of soot (‘bare’, ‘partly coated’ and ‘embedded’), we used only the particles for which we were able to clearly distinguish and measure the diameter of at least a couple of monomers. Only approximately 50% of all the images acquired for embedded soot particles were used for the calculation of D f . Supplementary Figs S3 and S4 show the fractal dimension of soot particles for each of the three categories based on coating: ‘bare soot’, ‘partly coated’ and ‘embedded’. Note that the number of particles in the ‘bare soot’ group is small, as only a small fraction of the total soot population was found to be bare (4%). In general, the data are more scattered in sample-1 than in sample-2. This variability is probably because the denuder was not kept at constant temperature during the collection of sample-1, resulting in particles with different degrees of denuding. How to cite this article: China, S. et al. Morphology and mixing state of individual freshly emitted wildfire carbonaceous particles. Nat. Commun. 4:2122 doi: 10.1038/ncomms3122 (2013).